Oncogenes create a unique landscape of fragile sites Recurrent genomic instability in cancer is attributed to positive selection and/or the sensitivity of specific genomic regions to breakage. Among these regions are fragile sites (FSs), genomic regions sensitive to replication stress conditions induced by the DNA polymerase inhibitor aphidicolin. However, the basis for the majority of cancer genomic instability hotspots remains unclear. Aberrant oncogene expression induces replication stress, leading to DNA breaks and genomic instability. Here we map the cytogenetic locations of oncogene-induced FSs and show that in the same cells, each oncogene creates a unique fragility landscape that only partially overlaps with aphidicolin-induced FSs. Oncogene-induced FSs colocalize with cancer breakpoints and large genes, similar to aphidicolin-induced FSs. The observed plasticity in the fragility landscape of the same cell type following oncogene expression highlights an additional level of complexity in the molecular basis for recurrent fragility in cancer. Genome instability is a hallmark of cancer. In early stages of cancer development, oncogene activation leads to replication stress [1] , [2] , [3] , [4] . Mechanisms by which oncogenes can induce replication stress include insufficient nucleotide pools to support extensive replication [4] , [5] , lack of other replication factors [6] and collision between replication and transcription [7] . In addition, a recent study showed that loss of FHIT expression encoded by the fragile histidine triad gene located in the fragile site locus FRA3B can initiate replication stress and continue genomic instability [8] . Regardless of the exact mechanism leading to replication stress, the stress results in the formation of DNA double strand breaks (DSBs) and genomic instability (reviewed by Hills and Diffley) [9] . Cyclin E and Ras are both known cellular oncogenes: overexpression of cyclin E or activating mutations in Ras such as G12V are found in many human cancers [10] , [11] , and lead to events of numerical instability, such as aneuploidy and polyploidy [12] , [13] , [14] . Additionally, oncogenic Ras expression [3] and overexpression of cyclin E induce replication stress, resulting in DNA DSBs and chromosomal rearrangements [4] . For both oncogenes insufficient nucleotide pools have been shown to be involved in the generation of replication stress [4] , [5] . Recurrent genome instability is attributed to positive selection and/or specific sensitivity of regions to breakage. Fragile sites (FSs) are specific genomic regions which appear as gaps, constrictions or breaks (referred to here as breaks) on metaphase chromosomes from cells grown under mild replication stress conditions. To date, most mapped FSs have been induced by low concentrations of aphidicolin, an inhibitor of the DNA polymerases α and δ [15] . An additional chemical inducer of FSs is hydroxyurea, an inhibitor of a key nucleotide biosynthesis gene, ribonucleotide reductase, which leads to low nucleotide pools and slow replication fork progression [16] . In the past, most FSs were mapped in lymphocytes. More recently, numerous aphidicolin-induced FSs have been shown to be cell type specific [17] , [18] , [19] . In human pre-cancerous lesions and following aberrant oncogene expression, genomic instability occurs preferentially at aphidicolin-induced FSs [2] , [4] . Breakage of aphidicolin-induced FSs in cancer cell lines and in pre-cancerous and cancerous samples is probably due to the inherent sensitivity of these regions to replication stress. Indeed, in many studies, comparisons were made between aphidicolin-induced FS and recurrent cancer instability. However, the cause of most recurrent genome instability in cancer remains unknown, since no association with recessive cancer genes or known lymphocytic aphidicolin-induced FSs has been reported [20] , [21] . Importantly, the lack of association between aphidicolin-induced FSs and cancer breakpoints can only partially be explained by the cell type-specific FSs [18] . Here we show that overexpression of cyclin E or mutated Ras in normal human fibroblasts leads to chromosomal breakage. Mapping the cytogenetic locations of the oncogene-induced FSs shows that in the same cells each oncogene creates a unique fragility landscape that only partially overlaps with aphidicolin-induced FSs. Oncogene-induced FSs share prominent features with aphidicolin-induced FSs such as colocalization with recurrent instability hotspots in cancer and colocalization with large genes. Altogether, our study reveals a novel complexity in the molecular basis for recurrent genomic instability in cancer and sheds light on the ability of transformation processes to change the sensitivity of regions to recurrent breakage. Oncogenes lead to chromosomal fragility We first examined whether overexpression of the oncogenes cyclin E and mutated H-Ras (H-Ras-V12, referred to henceforth as Ras) induces FS expression. To do so, BJ-hTERT cells were retrovirally infected with cyclin E, Ras or an empty vector (pbabe) as a control. Cyclin E and Ras overexpression was verified by Western blot ( Supplementary Fig. 1 ). After 2–8 weeks of cyclin E or 2.5 weeks of Ras overexpression, the cells were prepared for metaphase spread analysis. During this time cells cycled and proliferated constantly. To enable FS detection, we abrogated the G2/M checkpoint by adding a low concentration of the ataxia-telangiectasia mutated (ATM)/Rad3-related (ATR) inhibitor caffeine [22] . As can be seen in Fig. 1 , caffeine treatment alone resulted as expected in a very low level of total breaks. Treatment of caffeine together with low concentration (0.2 μM) of aphidicolin, commonly used to induce FSs, resulted as expected in a considerable level of total breaks. Importantly, cyclin E and Ras overexpression led to a significant total fragility compared with control cells treated with caffeine (two-sided Fisher’s exact test P =0.013 and 4.56E−08, respectively) and in some metaphases even resulted in chromosomal fragmentation ( Fig. 1 ). It is thus evident that overexpression of oncogenes can lead to FS expression that compromises chromosomal stability. 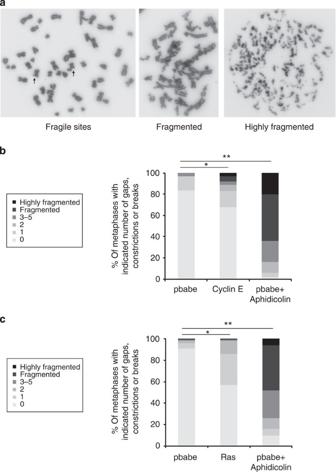Figure 1: General chromosomal fragility induced by cyclin E or Ras overexpression and aphidicolin treatment. (a) Examples of metaphases from BJ-hTERT cells overexpressing cyclin E and treated with 1.46 mM caffeine, showing different levels of chromosomal fragility. (b) Distribution of metaphases according to the level of chromosomal fragility in BJ-hTERT cells infected with empty vector (pbabe,n=97), cyclin E (n=100) and pbabe treated with 0.2 μM aphidicolin for 24 h (n=50). All cells were treated with 1.46 mM caffeine for 24 h.P-values are determined by two-sided Fisher’s exact test. *P<0.05;**P<3.5E−023. (c) Distribution of metaphases according to the level of chromosomal fragility in BJ-hTERT cells infected with empty vector (pbabe,n=98), Ras (n=100) and pbabe treated with 0.2 μM aphidicolin for 24 h (n=50). All cells were treated with 0.73 mM caffeine for 24 h.P-values are determined by two-sided Fisher’s exact test. *P<0.05**P<3.5E-023. Figure 1: General chromosomal fragility induced by cyclin E or Ras overexpression and aphidicolin treatment. ( a ) Examples of metaphases from BJ-hTERT cells overexpressing cyclin E and treated with 1.46 mM caffeine, showing different levels of chromosomal fragility. ( b ) Distribution of metaphases according to the level of chromosomal fragility in BJ-hTERT cells infected with empty vector (pbabe, n =97), cyclin E ( n =100) and pbabe treated with 0.2 μM aphidicolin for 24 h ( n =50). All cells were treated with 1.46 mM caffeine for 24 h. P -values are determined by two-sided Fisher’s exact test. * P <0.05; ** P <3.5E−023. ( c ) Distribution of metaphases according to the level of chromosomal fragility in BJ-hTERT cells infected with empty vector (pbabe, n =98), Ras ( n =100) and pbabe treated with 0.2 μM aphidicolin for 24 h ( n =50). All cells were treated with 0.73 mM caffeine for 24 h. P -values are determined by two-sided Fisher’s exact test. * P <0.05 ** P <3.5E-023. Full size image Specific repertoire of aphidicolin and oncogene-induced FSs Next, we investigated the repertoire of FSs induced by cyclin E and Ras overexpression and compared it with the repertoire of FSs induced in the same cells by aphidicolin. We mapped the chromosomal location of breaks on G-banded metaphase chromosomes from BJ-hTERT cells overexpressing cyclin E or Ras, and in cells infected with pbabe treated with low concentration (0.2 μM) of aphidicolin for 24 h. All cells were treated with 0.73 or 1.46 mM caffeine. A chromosomal locus was considered a FS if the number of breaks at that site accounted for at least 1% of the total breaks. The analysis of >300 breaks in each treatment revealed 24, 26 and 17 FSs in aphidicolin-treated, cyclin E and Ras overexpressing cells, respectively ( Fig. 2a–c and Supplementary Table 1 ). 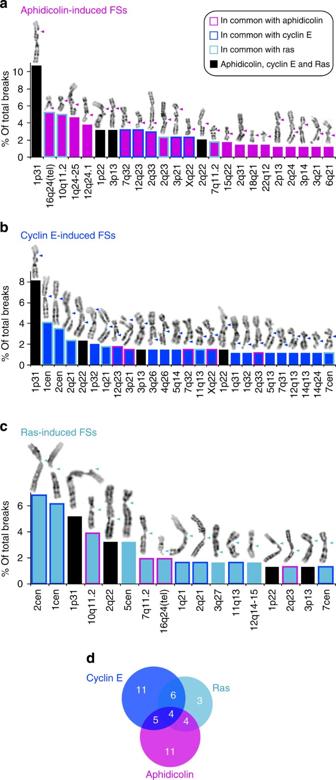Figure 2: Repertoire of aphidicolin and oncogene-induced FSs in human fibroblasts. Distribution of FSs identified on G-banded chromosomes of BJ-hTERT cells infected with (a) empty vector and treated with 0.2 μM aphidicolin for 24 h (b) cyclin E and (c) Ras. All cells were treated with 0.73 or 1.46 mM caffeine for 24 h. Breaks at indicated chromosomal bands are expressed relative to the total number of breaks (n>300). Representative examples for each FS are presented. (d) Overlap of the repertoires of FSs induced by aphidicolin treatment, cyclin E or Ras overexpression in BJ-hTERT cells. Figure 2: Repertoire of aphidicolin and oncogene-induced FSs in human fibroblasts. Distribution of FSs identified on G-banded chromosomes of BJ-hTERT cells infected with ( a ) empty vector and treated with 0.2 μM aphidicolin for 24 h ( b ) cyclin E and ( c ) Ras. All cells were treated with 0.73 or 1.46 mM caffeine for 24 h. Breaks at indicated chromosomal bands are expressed relative to the total number of breaks ( n >300). Representative examples for each FS are presented. ( d ) Overlap of the repertoires of FSs induced by aphidicolin treatment, cyclin E or Ras overexpression in BJ-hTERT cells. Full size image Comparison of the repertoire of FSs between cyclin E overexpressing and aphidicolin-treated cells revealed clear differences, as only 9/41 (22%) of the FSs were observed in both treatments ( Fig. 2a,b,d ). Remarkably, a difference in the repertoire of FSs is found even in the six most strongly induced FSs in each treatment, which include four FSs that are unique to aphidicolin (16q24, 10q11.2, 1q24-25 and 12q24.1) and four that are unique to cyclin E overexpression (1cen, 2cen, 2q21 and 1p32) ( Fig. 2a,b ). As in the case of cyclin E, Ras overexpression and aphidicolin treatment induced a different repertoire of FSs. Only 8/33 (24%) FSs appeared in both treatments: 9 FSs were induced only by Ras overexpression and 16 only by aphidicolin ( Fig. 2a,c,d ). Comparison of the FS repertoire between cyclin E- and Ras-overexpressing cells revealed that only 10/33 (30%) of the FSs ( Fig. 2b–d ) were induced by both oncogenes, out of which six were not induced by aphidicolin. In total, out of the total 44 FS regions found in either oncogene overexpression, or aphidicolin treatment, a substantial fraction (20 FSs, 45%) broke recurrently only upon oncogene overexpression and 11 FSs (25%) only upon aphidicolin treatment ( Fig. 2d ). Hence, 70% of the FSs showed condition-dependent fragility. As can be seen in Fig. 1b control cells (BJ-hTERT pbabe with 1.46 mM caffeine) have very low total breaks. A further analysis of 315 G-banded metaphases from control cells revealed only 56 breaks ( Supplementary Table 2 ). In comparison, in a similar number of metaphases from cyclin E (443 metaphases) and Ras (230 metaphases) expressing cells >300 breaks were identified. Most identified breaks in the control cells did not appear more than once. The repertoire of oncogene-induced FSs was enriched by recurrent fragility at the centromeres, which was not observed following aphidicolin treatment ( Fig. 2a–c ). However, one point that arises from the control cell analysis is that there are breaks located at centromeres. To investigate if cyclin E alone enhances centromeric fragility, we have analysed propidume-iodide (PI)-stained metaphases from BJ-hTERT cells infected with the control pbabe vector or the cyclin E vector, both with and without caffeine ( Fig. 3 ). The analysis shows that BJ-hTERT cyclin E cells have significantly more metaphases with fragile centromeres than BJ-hTERT pbabe cells, both with and without caffeine. This clearly shows that centromeric fragility is enhanced by cyclin E. This result is highly relevant to cancer development, since a substantial part of chromosomal aberrations in cancer involve centromeric/pericentromeric breakpoints [21] , [23] . 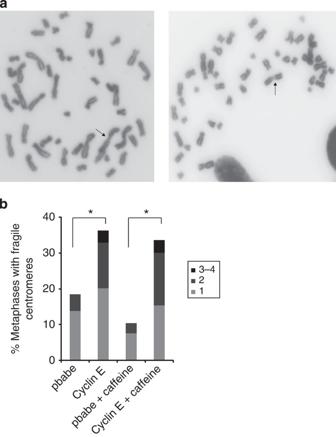Figure 3: Cyclin E enhances fragility of centromeres. (a) Examples of metaphases from BJ-hTERT cells overexpressing cyclin E without caffeine, showing fragile centromeres (indicated by arrows). (b) Percentage of metaphases with the indicated number of chromosomes showing fragile centromeres out of the total number of analysed metaphases in BJ-hTERT cells infected with empty vector (pbabe,n=152), cyclin E (n=149), empty vector with caffeine (n=145) and cyclin E with caffeine (n=143). Results are the summary of two independent experiments, on cells derived from one retroviral infection. Caffeine treatment is 1.46 mM caffeine for 24 h.P-values are determined by two-sided Fisher’s exact test. *P<0.005. Figure 3: Cyclin E enhances fragility of centromeres. ( a ) Examples of metaphases from BJ-hTERT cells overexpressing cyclin E without caffeine, showing fragile centromeres (indicated by arrows). ( b ) Percentage of metaphases with the indicated number of chromosomes showing fragile centromeres out of the total number of analysed metaphases in BJ-hTERT cells infected with empty vector (pbabe, n =152), cyclin E ( n =149), empty vector with caffeine ( n =145) and cyclin E with caffeine ( n =143). Results are the summary of two independent experiments, on cells derived from one retroviral infection. Caffeine treatment is 1.46 mM caffeine for 24 h. P -values are determined by two-sided Fisher’s exact test. * P <0.005. Full size image Importantly, out of the 56 identified breaks in the control cells only two sites (14q24 and 5q14) are mapped to the same site as recurrent non-centromeric oncogene-specific FSs. Hence, out of the 16 non-centromeric oncogene-specific FS ∼ 90% were not seen in the control cells. In summary, oncogene expression generates fragility in regions that are not sensitive to aphidicolin-induced replication stress in the same cells, and at the same time does not induce fragility in other aphidicolin-sensitive regions. This clearly indicates that upon oncogene overexpression a different repertoire of expressed FSs is generated in the same cells. Oncogene-induced FSs are recurrently deleted in cancer cells In order to further characterize oncogene-induced FSs we examined their colocalization with recurrent deletion clusters mapped in human cancer cell lines [20] . We found that 65% of the cyclin E as well as Ras-induced FSs coincided with a recurrent deletion cluster previously defined by Bignell et al . [20] as ‘unexplained deletion clusters’, because no association with known aphidicolin-induced FSs or recessive cancer genes was found ( Fig. 4a ). As Bignell et al . did not analyse centromeric regions, our centromeric FSs could not be analysed and thus were classified as ‘no data’ ( Fig. 4a ). Out of the aphidicolin-induced FSs mapped here in BJ-hTERT cells, 67% coincident with ‘unexplained deletion clusters’ ( Supplementary Fig. 3 ). This emphasizes that mapping of aphidicolin-induced FSs in any cell type, in addition to those mapped so far can explain additional deletion clusters found in cancer, as previously shown by Le Tallec et al . [18] . Notably, of the 29 FSs identified in our work that colocalize with previously unexplained deletion hotspots, 45% (13) are oncogene-induced FSs that are not induced by aphidicolin. These new findings highlight the complexity of defining FSs underlying recurrent fragility in cancer, as some FSs are induced by oncogenic overexpression and not aphidicolin ( Fig. 4b ). Furthermore, different oncogenes can create a unique landscape of FSs, even in the same cell type. 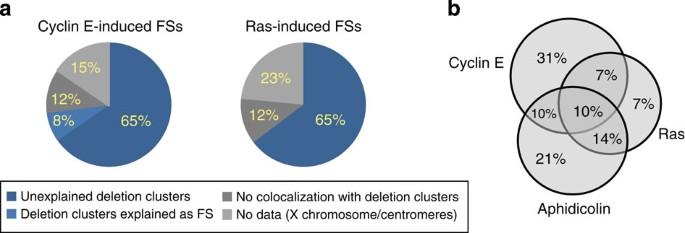Figure 4: Oncogene-induced FSs colocalize with recurrent deletion clusters in cancer cells. (a) Colocalization of the 26 and 17 FSs induced by overexpression of cyclin E and Ras, respectively, with recurrent deletion clusters in cancer cells published in Bignellet al.20(b) Colocalization of 29 FSs with unexplained deletion clusters (Bignellet al.) according to their mode of induction (expressed in %). Figure 4: Oncogene-induced FSs colocalize with recurrent deletion clusters in cancer cells. ( a ) Colocalization of the 26 and 17 FSs induced by overexpression of cyclin E and Ras, respectively, with recurrent deletion clusters in cancer cells published in Bignell et al . [20] ( b ) Colocalization of 29 FSs with unexplained deletion clusters (Bignell et al .) according to their mode of induction (expressed in %). Full size image Oncogene-induced FSs colocalize with large genes Another feature previously shown to be associated with many aphidicolin-induced FSs is colocalization with large genes (>300 kb) [18] , [24] . Gene content analysis revealed that similar to aphidicolin-induced FSs almost all (34/36 non-centromeric FSs) of the FSs induced by cyclin E or Ras colocalized with at least one large gene ( Fig. 5a , Supplementary Table 1 and Supplementary Fig. 4 ). 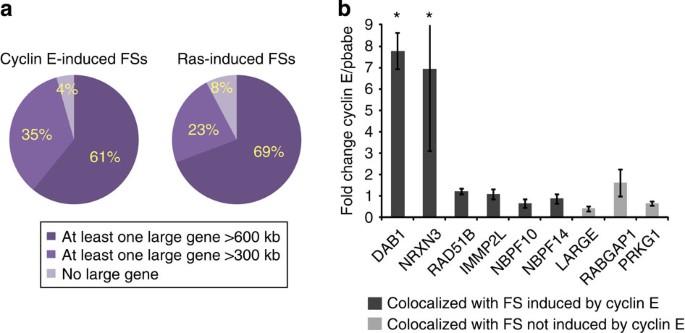Figure 5: Oncogene-induced FSs colocalize with large genes. (a) Colocalization of the 26 and 17 FSs induced by overexpression of cyclin E and Ras, respectively, with at least one large gene over the indicated length. (b) Fold change in expression of large genes (>600 kb) colocalized with FSs differentially expressed in BJ-hTERT cells overexpressing cyclin E or infected with empty vector (pbabe). Levels are mean fold change±s.e.m. (n⩾3).P-values are determined by paired two-tailed Studentt-test. *P<0.0004. Figure 5: Oncogene-induced FSs colocalize with large genes. ( a ) Colocalization of the 26 and 17 FSs induced by overexpression of cyclin E and Ras, respectively, with at least one large gene over the indicated length. ( b ) Fold change in expression of large genes (>600 kb) colocalized with FSs differentially expressed in BJ-hTERT cells overexpressing cyclin E or infected with empty vector (pbabe). Levels are mean fold change±s.e.m. ( n ⩾ 3). P -values are determined by paired two-tailed Student t -test. * P <0.0004. Full size image The transcription of large genes can lead to FS expression as a result of a collision between transcription and replication [25] , and oncogene overexpression can lead to transcriptional changes. Hence, we performed Real-time PCR on several very large genes (>600 kb) located within chromosomal bands harbouring FSs that differ in their expression between cyclin E and aphidicolin-treated cells. Two genes ( DAB1 , in 1p32 and NRXN3 in 14q24) showed a correlation between gene expression and fragility: gene expression was ∼ 7–8 fold higher in cyclin E-expressing cells compared with control cells in which no fragility is induced ( Fig. 5b ). In these cases, collision between transcription and replication could be the basis for the expression of the FS upon cyclin E overexpression. However, the expression level of seven other genes ( PRKG1, RABGAP1, LARGE, NBPF10, NBPF14, IMMP2L and RAD51B ) was similar with and without cyclin E overexpression ( Fig. 5b ). Furthermore, the expression level of five additional genes ( AUTS2, DCC, GPR98, GRM8 and FOXP2 ) was below detection level in all cells. These results suggest that a change in transcription of large genes is not the only mechanism explaining the observed variability in the FS landscape. In this study we revealed that oncogene expression induces fragile site expression and that the repertoire of FSs expressed in a given cell is extremely dynamic and dependent on the source of replication stress. Hence, the repertoire of aphidicolin-induced FSs only partially predicts the landscape of oncogene-induced FSs in the same cells. Moreover, different oncogenes lead to a different landscape of recurrent fragility. As different cancers involve overexpression of different oncogenes, our findings shed new light on the considerable variation of genomic aberrations observed between tumours originating from the same cell type [26] . Overall, the characterization of oncogene-induced FSs demonstrates that they share prominent features with aphidicolin-induced FSs such as colocalization with cancer genomic instability hotspots and large genes. Our results showing an overlap between oncogene-induced FSs and large genes further support the possibility that most large genes are actually FSs under specific replication stress conditions that were not yet discovered [18] , [27] . One interesting phenomenon enhanced by oncogene expression is fragile centromeres, which is not observed following aphidicolin-induced replication stress. Breakage at centromeres is highly relevant for cancer, as a study of thousands of cancer specimens found that in a typical cancer sample 25% of the genome is affected by chromosomal arm-level somatic copy-number alterations [21] . Our results showing recurrent fragility at centromeres on metaphase chromosomes before their segregation suggest that a pre-mitotic event can lead to chromosomal instability involving centromeres, such as losses or gains of whole chromosomes or chromosomal arms. Interestingly, a recent study revealed that replication-induced DSBs, rather than spindle defects, may lead to structural as well as numerical genomic instability [28] . Further studies are required to elucidate the mechanisms by which oncogenes enhance centromeric fragility, and whether the identity of the centromeres more prone to fragility is tissue specific, as observed for FSs. Generally, oncogene-induced fragility likely depends on the combination between the specific aberrantly expressed oncogene and the cell type in which it is expressed. Therefore, it will be interesting to investigate the FSs induced by oncogenes in cells originating from tissues in which the oncogene is aberrantly expressed, as for example cyclin E-induced FSs in ovarian, urothelial bladder and urothelial epithelial cells (although isolating such normal human cells is challenging). Transformation by oncogene overexpression could affect various processes which underlie the changes in the landscape of fragility. One effect of oncogene overexpression is transcriptional changes. In this study transcriptional changes of two large genes ( DAB1 and NRXN3 ) correspond to the change in the fragility of the FSs harbouring these genes (1p32 and 14q24, respectively). Other, yet undetermined, processes affected by oncogene overexpression could be epigenetic changes affecting, for example, the regulation of origins of replication. Abundance and initiation programs of origins of replications have been shown to set FS fragility [29] . Thus, changes affecting origin regulation and setting are likely to underlie changes in the landscape of fragility following oncogene overexpression. Since during tumour evolution cells continue to acquire genomic changes, including oncogene expression and tumour suppressor losses, due to instability and selection it is likely that plasticity in the repertoire of FSs takes place also in later stages of cancer development. To summarize, it has been suggested that recurrent deletions in tumours can be explained by the same FSs found by aphidicolin treatment of the tissue from which the cancer arises [18] . In light of our results showing that the FS landscape is different for different oncogenes in the same cell type, it is apparent that the recurrent fragility in cancer is more complex than previously appreciated. Future studies are required to elucidate the mechanisms by which oncogenes generate cellular changes that alter the sensitivity of genomic regions to replication stress. Cell culture and treatments Human foreskin fibroblasts BJ-hTERT cells (Clontech) were grown in DMEM supplemented with 10% foetal bovine serum, 100,000 U l −1 penicillin and 100 mg l −1 streptomycin. The cells were tested and found negative for mycoplasma. Aphidicolin and caffeine treatments were performed in growth media with the indicated concentrations. Retroviral infection Phoenix retroviral packaging cells were transiently transfected with vector plasmids. BJ-hTERT cells were infected three times with the Phoenix cell supernatant, which contained replication-defective viruses. Infected cells were then selected using 2 μg μl −1 of puromycin, for the next 10 days. Analyses were performed on one population of selected cells. For cyclin E and H-RAS-V12 overexpression, we used pbabe-puro-based vectors which were kindly provided by Professor J. Bartek and Professor D. Engelberg, respectively. Western blot analysis For protein separation, 10 and 15% polyacrylamide gels were used. The gel was transferred to a nitrocellulose membrane, and antibody hybridization and chemiluminescence were performed according to standard procedures. The primary antibodies used in this analysis were mouse anti-cyclin E (Leica NCL-cyclinE, 1:200), rabbit anti Ras (Santa Cruz SC-520, 1:6,000), mouse anti-Tubulin (SIGMA T5168, 1:50,000) and mouse anti-beta-Catenin (BD Transduction Laboratories 610153, 1:5,000). HRP-conjugated anti-rabbit and anti mouse secondary antibodies were obtained from Jackson Immunoresearch Laboratories (711-035-152 and 715-035-150, respectively, 1:5,000). Metaphase analysis Cells were treated with 100 ng ml −1 colcemid (Invitrogen, Carlsbad, CA, USA) for 15–40 min in incubator at 5% CO 2 . Then, cells were collected by trypsinization, treated with hypotonic solution at 37 °C for 30 min and fixed with multiple changes of methanol:acetic acid 3:1. Fixed cells were kept at −20 °C until analysis. For analysis of total gaps, constriction or breaks chromosomes were stained with propidume-iodide and blindly analysed. For cytogenetic mapping of FSs, chromosomes were classified according to the International System for Human Cytogenetic Nomenclature (ISCN), using the standard G-banding technique. RNA analysis Total RNA was extracted using the RNeasy extraction kit (QIAGEN). RNA-less and reverse-transcriptaseless reactions were used as controls. Complementary DNA (cDNA) synthesis was performed using the High Capacity cDNA Reverse Transcription Kit (Applied Biosystems). Real-time PCR was subsequently performed in AB 7300 using a Power SYBR green PCR master Mix (Applied Biosystems).The expression level was normalized to the transcript levels of POLR2A. Specific primers for these PCR reactions were designed using Universal ProbeLibrary assay design center (Roche) ( Supplementary Table 3 ). Statistical analysis For comparison of metaphases with chromosomal fragility and centromeric fragility (relevant to Figs. 1 and 3 ) two-sided Fisher’s exact test was used. For comparison of gene expression (relevant to Fig. 5b ) paired two-tailed Student t -test was used. How to cite this article : Miron, K. et al . Oncogenes create a unique landscape of fragile sites. Nat. Commun. 6:7094 doi: 10.1038/ncomms8094 (2015).